Multiscale cardiac modelling reveals the origins of notched T waves in long QT syndrome type 2 The heart rhythm disorder long QT syndrome (LQTS) can result in sudden death in the young or remain asymptomatic into adulthood. The features of the surface electrocardiogram (ECG), a measure of the electrical activity of the heart, can be equally variable in LQTS patients, posing well-described diagnostic dilemmas. Here we report a correlation between QT interval prolongation and T-wave notching in LQTS2 patients and use a novel computational framework to investigate how individual ionic currents, as well as cellular and tissue level factors, contribute to notched T waves. Furthermore, we show that variable expressivity of ECG features observed in LQTS2 patients can be explained by as little as 20% variation in the levels of ionic conductances that contribute to repolarization reserve. This has significant implications for interpretation of whole-genome sequencing data and underlies the importance of interpreting the entire molecular signature of disease in any given individual. The long QT syndrome type 2 (LQTS2) is an inherited arrhythmia syndrome in which mutations in the KCNH2 gene cause dysfunction of the rapid component of the delayed rectifying current ( I Kr ) resulting in delayed repolarization and the life-threatening ventricular arrhythmia torsades de pointes [1] . On the surface electrocardiogram (ECG), LQTS2 is characterized by prolongation of the QT interval and the appearance of ‘bifid’ or notched T waves [2] . The most thorough analysis of the mechanism of disease in LQTS2 showed that the vast majority (>90%) of missense mutants exerted their effect via reduced trafficking of proteins, resulting in decreased membrane conductance of I Kr (ref. 3 ). As such, LQTS2 represents one of the simplest arrhythmia syndromes with a well-described ECG phenotype. Despite this, predicting who is most at risk of lethal cardiac events is difficult, in part because of the great variability in presentation in relation to QT interval, the primary diagnostic criterion [4] . Furthermore, the origins of the notched T wave and its relationship with severity of the disease is not clear. Notched T waves have been included in diagnostic criteria for LQTS for the past 30 years [5] . They are also associated with poor prognosis in LQTS patients, although this empirical link was clouded by the mixed LQT genotype of the study population [6] . More recently, the prospect has been raised that more pronounced notching could represent more severe forms of LQTS2 (ref. 7 ). However, how I Kr dysfunction is related to notching of the T wave is not known and this has limited our ability to interpret the clinical significance of this ECG feature. The diagnostic puzzle for LQTS2 patients is further complicated by variability in the ECG phenotype. Population variability in the QT interval of LQTS patients has been previously reported [4] and linked to genetic variability [8] . This genetic underpinning may come in two guises. First, mutations of variable severity in a primary disease gene, that can be subclassified into those that reduce the membrane conductance of I Kr , either through disrupted trafficking or synthesis (the vast majority of cases [3] , [9] ) and those that alter the kinetics of I Kr current. Second, variants in other genes that contribute to repolarization reserve [10] might serve to modify the effect of a primary genotype [11] . In this regard, recent whole-exome sequencing studies have shown that genetic variation is extraordinarily extensive [12] , with every individual thought to have 20,000 variants in the coding regions [13] . The additive effects of these variants could explain both the variation in ECG phenotype in the LQTS2 population as well as the variable expressivity of primary LQTS2 disease genes, even within the same family [11] , [14] . Quantitatively analysing such a complex problem is far from trivial, however. For example, correlating many thousands of combinations of ion channel gene expression levels with variability in ECG characteristics is not practical by any conventional means. Furthermore, the electrical function of the heart is more than just the integrated activity of all the ion channels. The spread of electrical current from one region of the heart to another is influenced by myocyte connections, myofibre orientation and arrangement of muscle layers [15] and the overall geometry of the heart [16] . Not surprisingly then, it has been claimed that interrogation of such multivariable nonlinear dynamic systems necessarily involves the use of computer models [17] . In this study we have therefore used an in silico analysis to identify the origins of emergent ECG characteristics that we have observed in a LQTS2 patient cohort. We have previously employed a similar methodology in a simple multicellular system to conceptually address the question of whether ion channel expression levels might account for population variability in ECG phenotypes [18] . Until now, however, the extension of this approach to the intact ventricle, and hence the tackling of clinically useful questions, has been limited by the enormous computational burden of simulating many thousands of beats of the heart necessary to carry out such quantitative analysis. We have overcome this problem by harnessing a new high-performance computing paradigm, employing a supercomputer based on hardware normally reserved for graphics processing (graphic processing units, GPUs) to perform simulations of the heart [19] . We use this system to test the hypothesis that the population variability in gene expression within the rhythmonome has a significant impact on the variable phenotypic expression of LQTS2 patients. In doing so, we answer longstanding questions in regard to phenotypic presentation of LQTS2 including measuring a statistically significant correlation between the degree of T-wave notching and QT prolongation in a LQTS2 patient cohort, identifying the factors that contribute to notching of the T wave, quantifying how the effect of primary LQTS2 genotypes are modified by interperson variability in repolarization reserve and showing how additive genetic variability in the rhythmonome can account for variable expressivity of disease in LQTS2. T-wave notching in LQTS2 patients In addition to the pathognomonic feature of a prolonged QT interval, LQTS2 is typically associated with notching of the T wave ( Fig. 1a ). Among patients with LQTS2, there is however significant variation in both the extent of QT interval prolongation and the extent of T-wave notching. For example, in the Telemetric and Holter ECG Warehouse (THEW) cohort, the QT intervals (corrected for heart rate, QTc) were 520±45 ms for LQTS2 patients compared with 420±20 ms for controls ( Fig. 1b ). There was also variability in the extent of notching, which we found to be correlated with QTc (Spearman's Rank correlation; r =0.3, P <0.01, Fig. 1c ). To investigate the origins of notched T waves in LQTS2, we used an in silico approach. 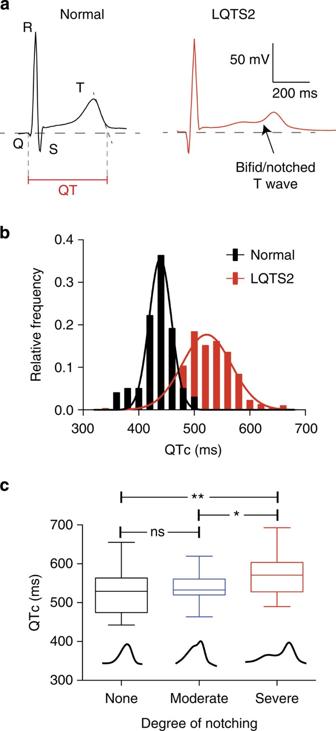Figure 1: Clinical characteristics of LQTS2. (a) Averaged beats at 1 Hz extracted from Holter ECGs of normal and LQTS2 patients. Examples shown are averages of >5,000 individual beats selected based on heart rate. The LQTS2 patient in this example was genotype positive for the Pro596Thr mutation inKCNH2. The major deflections of the ECG, designated Q, R, S and T waves are highlighted. QT interval for the averaged beats shown were 440 and 575 ms for normal and LQTS2, respectively, while notched T waves are evident only in the case of LQTS2. (b) Distribution of corrected QT intervals (QTc) in 158 normal (black) and 89 LQTS2 patients (red) measured from Holter ECGs. The mean QTcs were 420±20 and 520±45 ms for normal and LQTS2, respectively (s.e.m.). (c) Correlation of the degree of T-wave notching and QTc prolongation in LQTS2 patients. T-wave morphology was assessed in an averaged beat at 1 Hz extracted from Holter ECGs. Typical T-wave morphologies are shown for each category of patients. The mean QTc intervals for non-notched, moderate or severely notched T waves were 526±11 ms (s.e.m.;n=22), 539±8.7 ms (s.e.m.;n=24) and 571±12 ms (s.e.m.;n=22). *P<0.05, **P<0.01. Increasing degree of notching was correlated with QT interval (Spearman’s rank correlationr=0.3 (P<0.01)). Figure 1: Clinical characteristics of LQTS2. ( a ) Averaged beats at 1 Hz extracted from Holter ECGs of normal and LQTS2 patients. Examples shown are averages of >5,000 individual beats selected based on heart rate. The LQTS2 patient in this example was genotype positive for the Pro596Thr mutation in KCNH2 . The major deflections of the ECG, designated Q, R, S and T waves are highlighted. QT interval for the averaged beats shown were 440 and 575 ms for normal and LQTS2, respectively, while notched T waves are evident only in the case of LQTS2. ( b ) Distribution of corrected QT intervals (QTc) in 158 normal (black) and 89 LQTS2 patients (red) measured from Holter ECGs. The mean QTcs were 420±20 and 520±45 ms for normal and LQTS2, respectively (s.e.m.). ( c ) Correlation of the degree of T-wave notching and QTc prolongation in LQTS2 patients. T-wave morphology was assessed in an averaged beat at 1 Hz extracted from Holter ECGs. Typical T-wave morphologies are shown for each category of patients. The mean QTc intervals for non-notched, moderate or severely notched T waves were 526±11 ms (s.e.m. ; n =22), 539±8.7 ms (s.e.m. ; n =24) and 571±12 ms (s.e.m. ; n =22). * P <0.05, ** P <0.01. Increasing degree of notching was correlated with QT interval (Spearman’s rank correlation r =0.3 ( P <0.01)). Full size image Simulation of LQTS2 phenotype In the O’Hara–Rudy model of the human ventricular myocyte, a 50% reduction in I Kr produces 33% prolongation of the action potential measured at 90% recovery to baseline (APD 90 , Fig. 2b ). This correlated very well with the 31.8% prolongation of the QT interval seen in a heterogeneous cable representative of the transmural distribution of endocardial, midmyocardial and epicardial cells across the ventricular wall ( Fig. 2b ). Simulations of LQTS2 in the cable produced a slurred upstroke for the T wave but did not produce notching, consistent with previous observations from ourselves as well as other groups [20] , [21] , [22] . When we extended our simulations to the whole ventricle, which included cellular heterogeneity and details of tissue architecture (see Supplementary Fig. 3 ), the simulations produced both 30% prolongation of the QT interval and notched T waves. Conversely, simulations of LQTS3 ( Fig. 2f ) did not produce T-wave notching. In addition to these LQTS subtype-specific ECG phenotypes, our simulation system also reproduced clinically observed sex-specific differences in ECG parameters [8] based solely on knowledge of expression levels of ion channel genes [23] , thus further validating our in silico approach ( Supplementary Fig. 5 ). 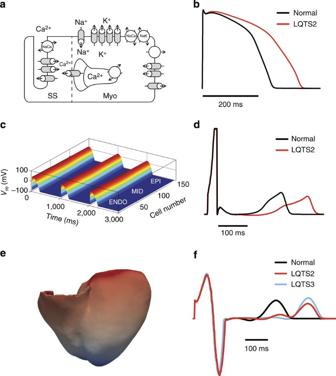Figure 2: Computational framework for simulation of LQTS2. (a) Schematic representation of a ventricular cell model37including membrane ion channels and pumps as well as intracellular calcium cycling. (b) Simulations of epicardial action potential waveforms for normal and LQTS2 (approximated by 50% reduction inIKrcurrent density). (c) Example of electrical propagation through a heterogeneous cable of 160 ventricular myocytes including endocardial, mid-myocardial and epicardial cells. (d) Pseudo-ECGs for normal and LQTS2 derived from the cable simulation shown in Bi. (e) Ventricular geometry used for simulation of ECGs. (f) ECGs derived from simulations of electrical propagation in the human ventricle for normal, LQTS2 and LQTS3. Simulated ECGs for LQTS2 and LQTS3 reproduce LQT subtype-specific ECG characteristics. Figure 2: Computational framework for simulation of LQTS2. ( a ) Schematic representation of a ventricular cell model [37] including membrane ion channels and pumps as well as intracellular calcium cycling. ( b ) Simulations of epicardial action potential waveforms for normal and LQTS2 (approximated by 50% reduction in I Kr current density). ( c ) Example of electrical propagation through a heterogeneous cable of 160 ventricular myocytes including endocardial, mid-myocardial and epicardial cells. ( d ) Pseudo-ECGs for normal and LQTS2 derived from the cable simulation shown in Bi. ( e ) Ventricular geometry used for simulation of ECGs. ( f ) ECGs derived from simulations of electrical propagation in the human ventricle for normal, LQTS2 and LQTS3. Simulated ECGs for LQTS2 and LQTS3 reproduce LQT subtype-specific ECG characteristics. Full size image Origins of notched T waves in LQTS2 In order to probe the genesis of notched T waves, we have aligned simulated ECGs ( Fig. 3a ) with an action potential (and its first derivative) from a cell located directly beneath the ECG electrode ( Fig. 3b ), and the major underlying ionic currents ( Fig. 3c ) for both the normal and LQTS2 simulations. The first peak in the LQTS2 bifid T wave is closely aligned to an initial minimum in the d V /d t of the AP waveform and the peak of I Kr (red-dashed line). This suggests that the membrane conductance of I Kr ( G Kr ) is a significant contributor to the first peak of the notched T wave (T1). The second component of the notched T wave is closely aligned with a second minimum in d V /d t and the peak of I K1 (dashed blue line). This is consistent with G K1 being the largest contributor to the second peak of the notched T wave (T2). Furthermore, the ‘well’ between T1 and T2 in LQTS2 is closely aligned with the peak of the reactivation of the sodium current (Cyan-dashed line) [24] . We suggest that in LQTS2, reduced G Kr leads to slowing of the rate of repolarization that results in cells spending a longer period of time in the voltage range where sodium channels reactivate (that is, the so-called I Na window current voltage range). This reactivation of the inward sodium current reinforces the slowing of repolarization and exacerbates the temporal deconvolution of the major components ( G Kr and G K1 ) of phase-three repolarization. It is also worth noting that in the normal heart there are still two minima in the cellular d V /d t trace (marked by the red and blue filled circles in Fig. 3b ), although they are not as well separated both in terms of amplitude and timing as that seen in LQTS2. 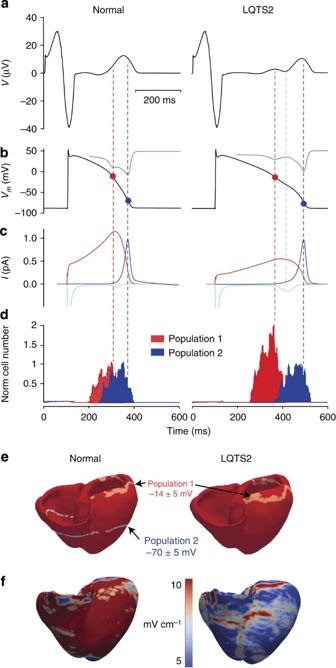Figure 3: Origins of T-wave notching in LQTS2. (a) Simulated ECGs for normal (left panel) and severe LQTS2 (right panel). (b) Action potential waveforms from an epicardial cell located directly beneath the recording electrode. Insets show the dV/dtfor each action potential waveform. The red and blue dashed lines indicate the two minima in the cellular dV/dt. A movie showing the spread of these repolarization phases for every cell from the heart are shown inSupplementary Movie 1. (c) Major ionic currents contributing to repolarization rate and bifid T waves in LQTS2.IKr(red),IK1(blue) andINa(cyan) are shown. Note that the red and blue dashed lines roughly correspond to the peak ofIKrandIK1, respectively. In the LQTS2 scenario, the peak of the window sodium current (dashed cyan line) corresponds to the trough in the notched T wave on the ECG. (d) The number of cells with voltages of −14±5 mV (population 1, red) and −70±5 mV (population 2, blue), corresponding to a 10-mV band around the two minima in cellular dV/dt, during the ECG. The peaks in the LQTS2 hearts are normalized to those observed in normal hearts. The temporal profiles of the two cell populations show significant overlap in the normal heart. Conversely, in LQTS2 hearts, population 1 is both significantly larger than in normal hearts and more clearly separated from population 2. (e) Images taken from the video inSupplementary Movie 1. Red and blue bands correspond to the repolarizing cell populations identified inb. In normal hearts the two populations are temporally coincident on the myocardium, while in LQTS2 hearts the bands are never coincident and hence contribute to individual components of the T wave. (f) Images taken from the video inSupplementary Movie 2, showing the spatial gradient of voltage at the time point corresponding to the red-dashed line ina–d. Whereas there is a smooth voltage gradient in the normal hearts, there is a more complex gradient in the LQTS2 hearts. Figure 3: Origins of T-wave notching in LQTS2. ( a ) Simulated ECGs for normal (left panel) and severe LQTS2 (right panel). ( b ) Action potential waveforms from an epicardial cell located directly beneath the recording electrode. Insets show the d V /d t for each action potential waveform. The red and blue dashed lines indicate the two minima in the cellular d V /d t . A movie showing the spread of these repolarization phases for every cell from the heart are shown in Supplementary Movie 1 . ( c ) Major ionic currents contributing to repolarization rate and bifid T waves in LQTS2. I Kr (red), I K1 (blue) and I Na (cyan) are shown. Note that the red and blue dashed lines roughly correspond to the peak of I Kr and I K1 , respectively. In the LQTS2 scenario, the peak of the window sodium current (dashed cyan line) corresponds to the trough in the notched T wave on the ECG. ( d ) The number of cells with voltages of −14±5 mV (population 1, red) and −70±5 mV (population 2, blue), corresponding to a 10-mV band around the two minima in cellular d V /d t , during the ECG. The peaks in the LQTS2 hearts are normalized to those observed in normal hearts. The temporal profiles of the two cell populations show significant overlap in the normal heart. Conversely, in LQTS2 hearts, population 1 is both significantly larger than in normal hearts and more clearly separated from population 2. ( e ) Images taken from the video in Supplementary Movie 1 . Red and blue bands correspond to the repolarizing cell populations identified in b . In normal hearts the two populations are temporally coincident on the myocardium, while in LQTS2 hearts the bands are never coincident and hence contribute to individual components of the T wave. ( f ) Images taken from the video in Supplementary Movie 2 , showing the spatial gradient of voltage at the time point corresponding to the red-dashed line in a – d . Whereas there is a smooth voltage gradient in the normal hearts, there is a more complex gradient in the LQTS2 hearts. Full size image At a tissue level, this deconvolution of phase-three leads to a greater apicobasal distribution of repolarization and the establishment of two distinct repolarizing populations across the myocardium in LQTS2. This can be represented most simply by quantifying the total number of cells in the heart that reside in the voltage bands (±5 mV) corresponding to the two repolarization phases identified in Fig. 3b throughout the time course of the ECG. In normal hearts, the temporal distributions of the two cell populations overlap ( Fig. 3d ) and are temporally coincident in the myocardium ( Fig. 3e and Supplementary Movie 1 ). As a result, they are integrated simultaneously into a monophasic T wave on the ECG. In LQTS2, the two repolarizing populations are temporally distinct ( Fig. 3d ) and as a result are never coincident in the myocardium ( Fig. 3e and Supplementary Movie 1 ). In the context of anisotropic conduction within the tissue, these distinct repolarizing phases establish complex spatial gradients of voltage that contribute to the notched T wave as well as potentially provide local steep voltage gradients that could be associated with re-entry ( Fig. 3e and Supplementary Movie 2 ). Molecular basis of phenotypic variability in LQTS2 We next turned our attention to the question: Why is there such phenotypic variability in LQTS2 (see Fig. 1b,c ). The first possibility we considered was that different mutations in the KCNH2 gene could result in different levels of I Kr dysfunction, either via reduction in I Kr membrane conductance ( G Kr ) or via altered I Kr kinetics. Since the vast majority (>90%) of LQTS2 mutants affect membrane conductance [3] , [9] , we first examined how alterations in I Kr density contributed to LQTS2 ECGs. In our simulations the extent of both QT prolongation and notching of the T wave increased as G Kr was reduced ( Fig. 4a,b ). However, while QT interval progressively increased, notching was only observed when G Kr was reduced by >30% ( Fig. 4b ). We also examined how alterations in I Kr kinetics contribute to ECG characteristics in LQTS2. The description of I Kr kinetics in the O’Hara cell model used in this study is based on Hodgkin–Huxley-type formulation, that is, a representation of macroscopic current characteristics not the molecular processes underlying conduction. This formulation allows us to incorporate simple changes to I Kr kinetics to examine in a general sense how changes that reflect altered voltage dependencies of activation/deactivation and inactivation of I Kr might differentially contribute to T-wave characteristics (Details in Supplementary Note 1 ). Simulated LQTS2 ECGs incorporating either defective trafficking, activation or inactivation of I Kr are shown in Fig. 4c . These simulations indicate that different mechanisms of I Kr dysfunction related to either trafficking or kinetics produce qualitatively similar changes to T-wave morphology; however, there are some subtle differences in terms of the timing and amplitude of T-wave peaks. This is not surprising, given the very different current profiles associated with each mechanism of dysfunction (See Supplementary Fig. 2 ). Analysis of the relationship between the severity of kinetic defects (represented by the magnitude of either the hyperpolarized shift in the voltage dependence of activation or the depolarized shift in the voltage dependence of inactivation) and ECG characteristics showed differential effects on QT prolongation and T-wave notching for each mechanism of kinetic dysfunction ( Fig. 4d–f and Supplementary Fig. 6 ). For example, increasing severity of inactivation defect affected T-wave morphology in a manner similar to reduced trafficking, showing a gradual prolongation of QT interval and T-wave notching that appeared with bigger shifts in the voltage dependence of inactivation. Conversely, changes to I Kr activation showed relatively little effect on either QT interval or notching with small shifts in the voltage dependence, but with more dramatic increases in both parameters with further activation defects. These differences in T-wave morphology associated with different mechanisms of I Kr dysfunction can be more simply illustrated by plotting the degree of notching or the time between T-wave peaks as a function of QT prolongation ( Fig. 4e,f ). Defects in I Kr activation cause more pronounced notching that occurs at shorter QT intervals compared with trafficking or inactivation-defective I Kr ( Fig. 4e ). Likewise, the time between T-wave peaks (T1–T2 time) is greater, at a given QT interval, in activation-deficient versus trafficking or inactivation-deficient I Kr ( Fig. 4f ). While the kinetic changes examined here are a simplistic representation of the myriad of molecular changes that could contribute to altered I Kr kinetics, they clearly demonstrate that LQTS2 mutations that cause changes in different kinetic properties of I Kr have potential to differentially modify the ECG compared with trafficking-defective mutants. Taken together, these data suggest that a variable reduction in I Kr density or function could be a significant contributor to variable expressivity of ECG phenotypes in LQTS2 patients. However, it cannot explain why members of the same family, with the same primary mutation, can also show significant variability in their phenotypes [11] , [14] . 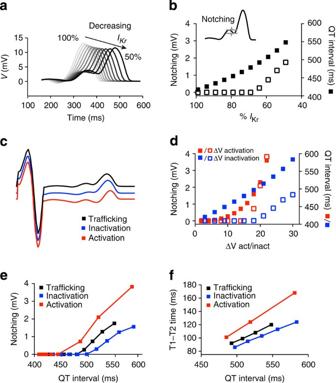Figure 4: Phenotypic severity of LQTS2 correlates withIKrdysfunction. (a) Magnified view of the T-wave component from simulated ECGs for stepwise reductions inIKrcurrent density (GKr) from 100 to 50%, representative of LQTS2 mutants that decrease protein trafficking. (b) Correlation between severity of trafficking defect and ECG characteristics for data shown ina. (c) Comparison of ECG waveforms resulting from impaired trafficking (45% reducedIKrcurrent density), a 21-mV hyperpolarized shift in the voltage dependence of inactivation and a 20-mV depolarized shift in voltage dependence of activation, which each prolonged the QT interval to ~520 ms. (d) Correlation between severity of kinetic defect and ECG characteristics. Voltage dependence forIKractivation was shifted between 2 and 24 mV in the depolarized direction, while the voltage dependence of inactivation was shifted between 3 and 30 mV in the hyperpolarized direction. (e,f) Relationship between QT interval and T-wave notching (e) and time between peaks of the notched T wave (T1–T2 time (f)) for LQTS2 ECGs representing trafficking, activation or inactivation defects. Figure 4: Phenotypic severity of LQTS2 correlates with I Kr dysfunction. ( a ) Magnified view of the T-wave component from simulated ECGs for stepwise reductions in I Kr current density ( G Kr ) from 100 to 50%, representative of LQTS2 mutants that decrease protein trafficking. ( b ) Correlation between severity of trafficking defect and ECG characteristics for data shown in a . ( c ) Comparison of ECG waveforms resulting from impaired trafficking (45% reduced I Kr current density), a 21-mV hyperpolarized shift in the voltage dependence of inactivation and a 20-mV depolarized shift in voltage dependence of activation, which each prolonged the QT interval to ~520 ms. ( d ) Correlation between severity of kinetic defect and ECG characteristics. Voltage dependence for I Kr activation was shifted between 2 and 24 mV in the depolarized direction, while the voltage dependence of inactivation was shifted between 3 and 30 mV in the hyperpolarized direction. ( e , f ) Relationship between QT interval and T-wave notching ( e ) and time between peaks of the notched T wave (T1–T2 time ( f )) for LQTS2 ECGs representing trafficking, activation or inactivation defects. Full size image To interrogate how the ECG presentation of a primary LQTS2 genotype can be modified by variable expression of other genes in the rhythmonome, we used a partial least squares (PLS) analysis (see Methods). This approach has not previously been experimentally tractable because of (a) the lack of pathogenic ECG features in simulations derived from simpler cellular arrangements (see Fig. 2 ) and (b) the immense computational load of generating the data sets required for sensitivity analysis of whole-heart electrical properties. For this part of the study, we used reduced I Kr current density (as opposed to altered kinetics) as the primary disease mechanism, since this is by far the most common cause of disease in LQTS2 (ref. 3 ). T waves from families of ECGs generated for normal hearts and moderate and severe LQTS2 are shown in Fig. 5a (right panel). Both the extent of prolongation and the variability of the QT interval increased with greater reductions in G Kr (407±7.5 ms at baseline, 454±8.6 ms for moderate LQTS2 and 534±11.5 ms for severe LQTS2 ( Fig. 5b )). T height on the other hand reduces and shows less variability with greater reductions in G Kr (12.4±0.4, 11.2±0.22 and 10.4±0.17 mV, respectively, Fig. 5c ). Measured parameters from these families of ECGs were then correlated with variation in the levels of individual ionic currents. The sensitivity matrix in Fig. 5d shows the relationships between the six most important membrane conductances in the cellular model and the three ECG parameters that define notching—the height of the two peaks of the T wave (T1 height and T2 height ) and the depth of the well between them (T1T2 depth ). It is clear that, first, there are significant differences in the contribution of each ionic conductance to individual determinants of notching and, second, individual ionic conductances contribute differently to different notched T-wave characteristics, that is, they have pleiotropic effects. The PLS regression allows quantification of these effects [18] , [25] ( Fig. 5e ). A PLS regression coefficient ( ρ ) of 0.69 for G Na and T1 height , for example, tells us that a 1-s.d. increase in G Na (5% in this case) results in a 0.69-s.d. increase in T1 height . The major determinants of T1 height are changes in G Kr and G Na ( ρG Kr =−0.59±0.07, ρG Na =0.69±0.03), while the major determinants of T2 height are G K1 and G Kr ( ρG K1 =+0.86±0.03, ρG Kr =−0.46±0.13). T12 depth is also primarily influenced by changes in G Kr , even in the background of already reduced G Kr in severe disease. These results correlate well with the currents identified as contributing to T-wave notching in Fig. 3 . Furthermore, the correlations between QTc and the extent of bifidness observed clinically ( Fig. 1c ) and in our simulations ( Fig. 4 ) are consistent with the PLS results, showing that changes in G Kr are the major contributors to both QTc and T12 depth . PLS analyses for all ECG parameters for normal and LQTS2 hearts are presented in Supplementary Figs 7–9 . 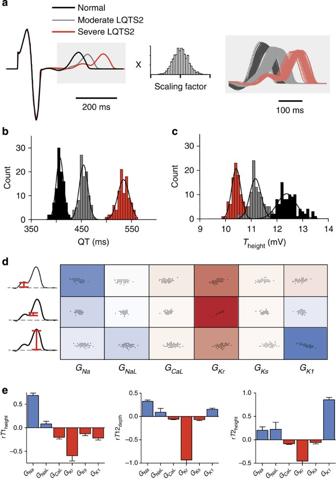Figure 5: Sensitivity analysis of the LQTS2 ECG. (a) Simulation pipeline for sensitivity analysis of the molecular basis of T-wave notching. Ionic conductances in the cellular model defining the baseline ECG were modified according to a log-normal distribution of randomized scaling factors with a s.d. of 5%. This process was repeated 100 times for each genotype to yield families of ECGs for normal, moderate LQTS2 and severe LQTS2. Moderate and severe LQTS2 were approximated by 25 and 50% reduction inGKr,respectively. (b,c) Distributions of QT interval (b) and Theight(c) as a function of severity of LQTS2. (d) Sensitivity matrix showing the relationship between the three main ECG characteristics defining T-wave notching (height of the first peak of the T wave (T1height), depth of the well between T-wave peaks (T1T2depth) and height of the second peak of the T wave (T2height)) and the six most important membrane conductances (Gx). The scatter plots in each panel describe the relationship between variability in expression/conductance of a particular ion channel and variability in an ECG parameter. Each data point in the scatter plots represents an individual measurement from the families of ECGs ina. Panels are coloured according to magnitude and sign of the correlation in the scatter plot. (e) Partial least squares regression of data fromdquantifying the sensitivity of T1height(left panel), T12depth(centre panel) and T1height(right panel) to variability in individual ionic conductances. Values are mean±s.d. from three independent sets of simulations. Figure 5: Sensitivity analysis of the LQTS2 ECG. ( a ) Simulation pipeline for sensitivity analysis of the molecular basis of T-wave notching. Ionic conductances in the cellular model defining the baseline ECG were modified according to a log-normal distribution of randomized scaling factors with a s.d. of 5%. This process was repeated 100 times for each genotype to yield families of ECGs for normal, moderate LQTS2 and severe LQTS2. Moderate and severe LQTS2 were approximated by 25 and 50% reduction in G Kr, respectively. ( b , c ) Distributions of QT interval ( b ) and T height ( c ) as a function of severity of LQTS2. ( d ) Sensitivity matrix showing the relationship between the three main ECG characteristics defining T-wave notching (height of the first peak of the T wave (T1 height ), depth of the well between T-wave peaks (T1T2 depth ) and height of the second peak of the T wave (T2 height )) and the six most important membrane conductances ( G x ). The scatter plots in each panel describe the relationship between variability in expression/conductance of a particular ion channel and variability in an ECG parameter. Each data point in the scatter plots represents an individual measurement from the families of ECGs in a . Panels are coloured according to magnitude and sign of the correlation in the scatter plot. ( e ) Partial least squares regression of data from d quantifying the sensitivity of T1 height (left panel), T12 depth (centre panel) and T1 height (right panel) to variability in individual ionic conductances. Values are mean±s.d. from three independent sets of simulations. Full size image Variable expressivity of LQTS2 genotypes We next wanted to test the hypothesis that additive changes in expression of multiple modifier genes could explain the variable expressivity observed in LQTS2, where patients with the same primary gene defect show significantly different ECG presentations. As an example, Fig. 6a shows averaged beats at 1 Hz from Holter ECGs recorded from two female patients, aged 20 and 24 years, with the same LQTS2 mutation (D501N, a mutant that we have characterized as trafficking-defective ( Supplementary Fig. 10 )), but very different ECG phenotypes (black trace: monophasic T wave, red traces: notched T wave and more markedly prolonged QT interval). To address this question, we simulated ECGs reflecting all possible combinations of baseline and ±10% conductance levels of the three non- G Kr conductances ( G K1 , G Na and G CaL ) that contributed most to T-wave notching (from Fig. 5e ). This gives a total of 3 3 , or 27, different combinations of expression levels, for which we then simulated ECGs (each equilibrated for 200 beats at 1 Hz). We measured ECG parameters from each of these simulations and used them to construct ‘wheel of fortune’ plots [18] , [26] to represent the relationship between combinations of altered ion channel expression levels and notched T waves on the ECG ( Fig. 6b,c , Supplementary Fig. 12 ). In these plots, each of the 27 segments represents one of the possible combinations of conductance level variation in our three selected ion channels coloured according to the level of conductance (black: +10%, grey: baseline, white: −10%). In each plot, the combinations are sorted according to the magnitude of the measured parameter, from highest (red, at the 2 o’clock position) to the lowest (blue, at the 10 o’clock position). The concentration of black segments (+10%) to the right and white segments (−10%) to the left in the G Na band for T1 height indicates that in the context of reduced G Kr , changes to G Na are the major determinants of T1 height . For example, a 10% increase in G Na combined with a 10% decrease in G Cal and G K1 increases T1 height from 2.6 μV at baseline to 3.3 μV ( Fig. 6b ). Conversely, changes in G K1 clearly have the major influence on T2 height ( Fig. 6c ). It is also worth noting that the patterns of conductance combinations that modify the ECG are different for each component of the T wave (see also Supplementary Fig. 12 ). 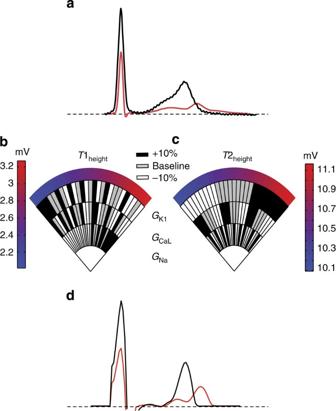Figure 6: Additive effects of multiple genetic variants can explain variable expressivity in LQTS2. (a) Examples of variable expressivity of LQTS2. Averaged ECG traces from 5 s of Holter ECG recordings from two patients with the same D501N LQTS2 mutation are shown. Data were taken during sleep at 0300 hours to remove confounding effects of circadian rhythm and variable adrenergic tone. Patient 1, a 24-year-old female (black trace), has a QTc of 538 ms (corrected using Fridericia’s correction formula43) and a non-bifid T wave, while patient 2, a 20-year-old female (red trace), has a QTc of 585 ms and a bifid T wave. The D501N mutation results in ~50% reduction in protein trafficking (seeSupplementary Fig. 10). (b,c) ‘Wheel of Fortune’ plots showing epistatic modification of T1height(a) and T2height(b) byGNa,GCaLandGK1in a background of a 40% reduction inGKr. (d) Simulated ECGs starting withGKrat 62.5% and then modified according to the wheels of fortune to minimize bifidness (black: decreasedGNa, increasedGKr,GCaLandGK1) and maximize bifidness (red: increasedGNa, decreasedGKr,GCaLandGK1). Figure 6: Additive effects of multiple genetic variants can explain variable expressivity in LQTS2. ( a ) Examples of variable expressivity of LQTS2. Averaged ECG traces from 5 s of Holter ECG recordings from two patients with the same D501N LQTS2 mutation are shown. Data were taken during sleep at 0300 hours to remove confounding effects of circadian rhythm and variable adrenergic tone. Patient 1, a 24-year-old female (black trace), has a QTc of 538 ms (corrected using Fridericia’s correction formula [43] ) and a non-bifid T wave, while patient 2, a 20-year-old female (red trace), has a QTc of 585 ms and a bifid T wave. The D501N mutation results in ~50% reduction in protein trafficking (see Supplementary Fig. 10 ). ( b , c ) ‘Wheel of Fortune’ plots showing epistatic modification of T1 height ( a ) and T2 height ( b ) by G Na , G CaL and G K1 in a background of a 40% reduction in G Kr . ( d ) Simulated ECGs starting with G Kr at 62.5% and then modified according to the wheels of fortune to minimize bifidness (black: decreased G Na , increased G Kr , G CaL and G K1 ) and maximize bifidness (red: increased G Na , decreased G Kr , G CaL and G K1 ). Full size image Using these ‘wheel of fortune’ plots to guide the choice of conductance variations, we investigated whether we could reproduce the clinical variability we observed in Fig. 6a . Starting with 62.5% G Kr as a baseline for our simulations, we added variability of up to ±20% for each of the ionic conductances in the cell and were able to reproduce all of the trends seen in the patient example ( Fig. 6a ). The specific conductance levels used to generate the ECGs shown in Fig. 6d are detailed in Supplementary Table 1 . These results suggest that 20% or less variation in levels of ion channel expression could explain the variable expressivity in both QT interval as well as T-wave morphology observed in patients with LQTS2. In this study we report a correlation between notched T-wave morphology and QT prolongation in LQTS2 patients. Furthermore, using an in silico approach based on a novel GPU-based simulation environment we have identified the ionic currents and cellular properties that determine this signature ECG phenotype and quantified how multiple small genetic hits can account for the variable ECG patterns in this disease. It is well established that the bifid, or notched, T wave is a ‘signature’ characteristic of LQTS2 (ref. 2 ); however, the correlation with QT interval, the current primary diagnostic measure, has not been made previously. While earlier studies have raised the possibility that notched T waves correlate with worse prognosis, notching was not well correlated with QT prolongation in patients with symptomatic LQTS [6] , [27] . However, these observations were made in the pre-genotype era, meaning the mixed genotype of the study populations (that is, many of the symptomatic patients would have had LQTS1 or LQTS3) would confound any LQTS subtype-specific correlations. In our study, we were able to measure a statistically significant correlation by extracting beats from Holter recordings under similar conditions (for example, just comparing beats at heart rates of 60 b.p.m., during the night) to permit a genuine like-for-like comparison between patients (see Supplementary Fig. 1 ). Our simulations based on the O’Hara ventricular cell model showed that both of these phenomena, QT prolongation and T-wave notching, are related to the degree of I Kr dysfunction. T-wave notching was observed in simulations regardless of whether the mechanism of I Kr dysfunction was related to protein trafficking or altered kinetics of I Kr . However, it was clear that defects related to different kinetic processes defined subtly different notched profiles in our simulations. In particular, defects in I Kr activation caused more pronounced notching and more significant separation of T-wave peaks than inactivation or trafficking defects that caused a similar degree of QT prolongation. In all cases, however, notching of the T wave was only observed with more substantial dysfunction of I Kr . This indicates that a significant disruption of the repolarization reserve is necessary for T-wave notching to be manifested, and suggests this may be a useful indication of more severe disease in LQTS2. In the clinic, notched T waves are almost exclusively observed in patients with LQTS2 (ref. 2 ), and indeed in our simulations of LQTS3 we did not observe T-wave notching. Our data showing that the extent of notching is related to the extent of decrease in I Kr provide the first plausible mechanistic insight into the origin of notched T waves and explains why they are primarily associated with LQTS2. Simulation of cardiac electricity is an extremely useful tool that allows interrogation of the electrical environment of the heart in ways that are too complex to tackle using conventional physiological techniques. Recently, several groups including ourselves have used sensitivity analysis at the level of individual cells [28] , [29] or in simple multicellular systems [18] to evaluate how differential expression of cardiac ion channels results in interperson variability in ECG parameters. However, because of the problem of computational load, it has not been possible to tackle this problem at the organ level. To overcome this hurdle, we developed a highly parallelized implementation of the Cancer, Heart and Soft Tissue Environment [30] utilizing General Purpose computing on GPUs (GPGPU). Parallel computing exploits the fact that a large problem can be subdivided into many smaller ones that are solved simultaneously, conventionally by distributing the sub-problems to CPU-processing ‘cores’ on interconnected computers. GPGPU takes advantage of the architecture of GPUs that are highly optimized for the parallel data-processing requirements of computer graphics. Each GPU contains many hundreds of processing cores and, furthermore, many GPUs can be connected together, allowing very high degrees of parallelization to be achieved (many thousands of parallel calculations) without the overhead of data transfer between computers. Other groups have already demonstrated the value of the GPGPU approach for simulation of cardiac electrical activity [31] , [32] . Our approach of using a GPU-based supercomputer to parallelize not only the simulation of individual hearts but also the simulation of hundreds of concurrent instances is the technological advance that makes our analysis possible ( Supplementary Fig. 13 ). The GPGPU implementation of Chaste that we have developed in this study will enable the wider community to tackle other problems in cardiac and cancer physiology that have to date been limited by computational scale. Over the last 20 years, great progress has been made in identifying the molecular causes of inherited arrhythmia syndromes; yet we still do not know how perturbations in these components are linked through the web of interactions between molecules, cells and tissues, to observed clinical phenotypes [2] . Our simulations of the human ventricle were able to reproduce the notched T waves observed in LQTS2 and therefore allow the investigation of the origin of this phenomenon for the first time. In a previous study based on the canine wedge preparation [33] , the appearance of notched T waves was only seen when I Kr was reduced by a combination of sotalol (an I Kr blocker) and hypokalaemia. They concluded that the notching was caused by delayed repolarization in M cells. This study however was precluded by the nature of the tissue preparation from addressing the contribution of whole-heart properties; for example, the contributions of apicobasal gradients that are also thought to influence T-wave morphology. Furthermore, the question of whether these transmural voltage gradients related to midmyocardial cells exist in the intact heart, and hence contribute to the T-wave morphology, is a matter of some debate [34] , [35] . Our studies extend this observation by highlighting that the slowing of repolarization has to be in the critical range of voltages that permits more extensive reactivation of the sodium channel window current, which in turn amplifies the deconvolution of the major components of phase-three repolarization. More specifically, the major contributors to phase-three repolarization in the resting heart ( G Kr and G K1 ) are sufficiently temporally separated in LQTS2 that over the time period of apex to base conduction form separate repolarizing populations that contribute to the individual peaks of the notched T wave. Furthermore, by using a PLS analysis we have shown that not only is notching a complex function of multiple ionic conductances but also that each conductance can have pleiotropic effects on the T wave. For example, increasing G K1 decreases the height of the first component of the bifid T wave (T1 height ) and increases the height of the second component (T2 height ). Our analysis therefore demonstrates that T-wave morphologies associated with disease are complex functions of molecular, cellular and tissue level properties of the heart and that notching of the T wave is correlated with severity of LQTS2 with the exact morphology is fine-tuned by other ion channels that contribute to repolarization reserve. In our analysis of LQTS2 patients, we observed, as other have previously [4] , that there is significant variability in the clinical presentation, specifically in regard to their QT interval (see Fig. 1b ). More strikingly, even patients with the same primary genotype can have significantly different disease phenotypes, varying from severe to largely asymptomatic (ref. 11 and Fig. 6a ). There are many factors that can potentially contribute to this variable presentation, including differences in autonomic tone, variability in the level of hormones that modify cardiac electrical activity as well as age, sex and body habitus. In our example of variable expressivity ( Fig. 6a ), we sought to minimize these effects where possible by using an example of age- and sex-matched individuals, with representative beats extracted from their Holter recordings at 1 Hz during the night to minimize the confounding effects of autonomic tone. The hypothesis that we tested in this study to explain this phenotypic variability is that the additive effects of variable expression in the genes coding for other ion channels that contribute to the repolarization reserve can modify the effect of the primary mutation, and hence the phenotypic presentation [11] . It is far from trivial, however, to quantify the contribution of these small effect variants, and very large studies are required to quantify the effects of even one of them. As a result, quantitative analysis of the combinatory effects of multiple modifying variants, which in all likelihood are present in every patient based on recent analysis of the frequency of single-nucleotide polymorphisms in the population [12] , is all but impossible by conventional means. However, by using the computational framework presented in this study we have been able to address this question in silico . Our analysis suggests that in patients with the same primary genotype the presence or absence of a notched T wave could be accounted for by as little as 20% variation in the levels of other ion conductances. These data therefore show how small effect genetic variants can account for variable expressivity of primary disease mutations, even within the same family and explain the apparently low penetrance of many LQTS2 mutations [11] , [14] . The analysis also demonstrates that consideration of multiple parameters related to morphology of the T wave provides much greater discrimination of the impact of both individual variations as well as combinations of variants. In summary, we have reported a correlation between the degree of notching of the T wave and QT prolongation in LQTS2 patients and identified the origins of this signature ECG phenotype. Our method hinged on development of a novel computational framework, allowing us to simulate the hundreds of thousands of heartbeats necessary to quantitatively analyse the basis of emergent properties of the ECG. Using this approach we have been able to elucidate the pleiotropic effects of ion channel expression variability on the cardiac ECG as well as modification of disease phenotypes by second, third or more genetic hits. In addition to these specific insights, the multiscale modelling that we have been able to employ to interrogate the causal relationships between low-level inputs (that is, variability in membrane conductance of cardiac ion channels) and emergent properties of an organ-level system demonstrates the potential for analysis of whole-organ function in other disciplines of physiology and medicine. The ventricular geometry employed in this study does not contain a conduction system, meaning our study was limited to ECG parameters related to repolarization rather than activation of the myocardium. In relation to our analysis of the affects of altered I Kr gating on the ECG, the model of I Kr used in the O’Hara–Rudy ventricular cell model is a Hodgkin–Huxley-type description of macroscopic current. As a result, we are unable to examine how LQTS2 mutants that affect the molecular processes underlying specific gating processes contribute to the ECG. Future studies incorporating molecularly accurate Markov descriptions of hERG gating will no doubt shed greater light on the contribution of altered I Kr gating to LQTS2 ECGs. Patient cohorts Holter ECGs were obtained through collaboration with the THEW [36] . The normal patient cohort consisted of 202 24-hHolter recordings from patients without cardiovascular diseases. The LQTS data set consists of 480 24-h Holter recordings (145 LQTS2) from 307 genotyped patients. Holter recordings were processed using an automated beat averaging routine to identify segments of the trace that had a stable HR close to 60 b.p.m. Averaged beats from these regions were then analysed using an ECG-processing software developed in house (see Supplementary Fig. 1 ) and quality controlled by a trained cardiologist. T waves were classified as non-notched, moderate or severely notched by three independent blinded reviewers. Cell culture and transfections Human embryonic kidney cells (HEK293, European Cell Culture Collections) were maintained in culture in Dulbecco’s modified Eagle medium nutrient mixture F-12 (Ham; DMEM/F-12; Gibco) supplemented with glutamax and 10% fetal calf serum. Cells were transiently transfected with C-terminal HA-tagged wild-type or D501N Kv11.1 cDNA in pIRES2eGFP (Clonetech), using Lipofectamine 2000 (Life Technologies). Cells were harvested 40 h after transfection and lysed for SDS–PAGE and subsequent western blot analyses. Nitrocellulose membranes were probed simultaneously with a mouse monoclonal anti-HA antibody (Covance, Princeton, NJ, USA) using 1:20,000 dilution and rabbit anti-α-actinin antibody at 1:1,000 dilution (Cell Signaling Technology, Danvers, MA, USA) followed by anti-mouse IRDye800 and anti-rabbit IRDye680 antibodies (Li-Cor Biotechnology, Lincoln, NE, USA), both at 1:20,000 dilution. The membrane was scanned on a Li-Cor Odyssey system to quantify the relevant protein bands using Image Studio (Version 4). Uncropped scans of the western blots are provided in Supplementary Fig. 11 . Ventricular cell model Membrane biophysics was described using the O’Hara ventricular model of epi-, endo- and midmyocardial cells [37] . This cellular model was chosen, since it is based entirely on data from healthy human tissue. The sodium channel in the O’Hara model was replaced with the Markov description of Nav1.5 from Clancy and Kass [38] to enable incorporation of LQTS3 mutant genotypes that resulted in a non-inactivating component of the sodium current ( I Na ). The new I Na description was scaled such that peak current amplitudes during the AP were unaltered. Recent results suggest that Nav1.8 is responsible for the late sodium current in cardiomyocytes [37] , [39] . We therefore left the existing persistent sodium current of the model unaltered. Within the cellular model, each current component ( I x ) is defined such that: where G x is the maximal conductance, P o x is the open probability and E rev is the reversal potential. Variability to membrane conductance was implemented through the addition of scalars to the conductance parameter ( G x ). For simulations including altered I Kr kinetics, parameters relating to the voltage dependence of activation and inactivation gating were modified as detailed in the Supplementary Note . Structural mesh Simulations were carried out in a tetrahedral meshed representation of the left and right ventricles of the human heart obtained from the Chaste group at the Oxford University, UK (freely available to download at http://www.cs.ox.ac.uk/chaste under the BSD license) [40] . The mesh consisted of 714,459 elements resulting in 137,483 nodes at an average spacing of 1.2 mm. Tissue heterogeneities including fibre orientation and transmural distributions of epi-, endo- and midmyocardial cells were included in the tissue description (see Supplementary Fig. 3 for details). Electrical propagation/ECG calculation All simulations were carried out on a GPGPU implementation of Chaste [30] developed in house and deployed on the 'Bragg' GPU supercomputer (CSIRO, Australia). The differential equation used to describe electrical propagation in our human ventricular tissue is: where χ is the surface area-to-volume ratio (1,400 cm −1 ), C m is the specific membrane capacitance (1 μF cm 2 ), u is state variable vector defined by cell model equations, σ is an effective conductivity and I stim is a stimulus current applied at the ventricular apex (2 ms duration, 80 mA cm −3 ) [41] . Bulk conductivity tensors were implemented resulting in conductivities of 7 mS cm −1 along myofibres, 3.5 mS cm −1 transverse to myofibres but in the plane of myolaminae, and 1.6 mS cm −1 normal to myolaminae [15] . An explicit time integration scheme, with time steps of 0.005 and 0.1 ms, was used in solution of cellular ordinary differential equations and the partial differential equation, respectively. Pseudo-ECGs were calculated according to the equation: where ∇ V m is the spatial gradient of voltage and r is the distance from a source point ( x , y , z ) to a field point ( x ′, y ′, z ′) [42] . In all experiments, ECGs were derived using an electrode placed 2 cm from the epicardial surface of the left ventricle. GPU simulation environment All simulations were performed on the CSIRO Accelerator Cluster (Bragg). The Bragg cluster consists of 128 Dual Xeon 8-core E5-2650 Compute Nodes each with 128 GB of RAM and FDR10 InfiniBand interconnect. GPU resources on the Bragg cluster comprise 132 Fermi Tesla M2050 GPUs (a total of 59,136 CUDA cores) and 254 Kepler Tesla K20 GPUs (a total of 633,984 CUDA cores). To confirm the accuracy of our GPU-based implementation of Chaste, the wild-type model was simulated for 2 s of output and the results compared with the same simulation scenario implemented on the standard CPU-based version of Chaste. The two simulations were identical. Our GPU implementation of Chaste will be available in future software versions. A virtual machine pre-installed with GPU-Chaste (capable of simple proof-of-principle simulations) together with a Matlab workspace containing all data and simulation outcomes used in this study are available at www.victorchang.edu.au/Hill_Lab . PLS analysis To assess the sensitivity of ECG parameters to changes in individual ionic currents in the cardiac myocyte, we employed the PLS analysis [25] . This technique correlates the effects of variation of input parameters of a model (ionic conductances through channels and pumps) with output parameters (such as QT interval, T1 height and so on). For each instance of the PLS analysis, the system was solved for 100 different scenarios. In each scenario, all conductance parameters in the model ( G x from equation 1) were individually scaled by a random number drawn from a log-normal distribution centred around a mean value of 1, with s.d. of 5%. A single scaling factor was applied to each conductance across the entire heart, regardless of whether the particular conductance varied depending on cell type (that is, epi- mid- and endocardial cells). For every scenario, the system was equilibrated for 200 beats after parameter randomization to account for long-term changes in ionic concentrations (see Supplementary Fig. 4 ). After equilibration, ECG parameters were measured from the 200th beat and saved with the corresponding set of randomized scaling factors. Matrices containing ECG parameters and scaling factors were log-transformed, centred on their mean values and normalized to their means. These values were used as inputs for the PLS function PLSREGRESS in the Matlab Statistics Toolbox (Mathworks, MA, USA). The output of this function is an array of PLS regression coefficients ( ρ ) that describes the model’s sensitivity for each ionic conductance. To get an estimate of error in PLS regressions, data sets of 100 simulations were randomly split into three groups and PLS analysis was carried out on each sub-data set. The means and s.d.’s of PLS coefficients were derived from the three outputs. Wheel of fortune plots To generate ‘Wheel of Fortune’ plots [18] , [26] , we examined three ionic conductances in each case. Each of these conductances were varied by ±10%, which, together with the baseline level, gives a total of 3 3 (three levels of three different conductances) or 27 different combinations for each plot. For each of these 27 combinations, we simulated ECGs (each equilibrated for 200 beats at 1 Hz). ECG parameters measured from these simulations were used to generate the ‘genetic wheel of fortune’ plots. In each plot, each of the 27 segments represents one of the possible combinations of conductance level variation in our three selected ion channels shaded according to the conductance level such that the baseline level of each conductance is shown in grey, an increase of 10% in white and a decrease of 10% in black. Combinations are then sorted according to the magnitude of the measured parameter shown in the outer ring of the plots colour-coded from the highest (red) to the lowest (blue). A 40% reduction in G Kr was chosen as the background for these simulations, since in more severe LQTS2 (that is, 50% G Kr reduction) many of the epistatic modification scenarios precipitated breakdown of regular activity and so useful parameters could not be extracted. How to cite this article: Sadrieh, A. et al . Multiscale cardiac modelling reveals the origins of notched T waves in long QT syndrome type 2. Nat. Commun. 5:5069 doi: 10.1038/ncomms6069 (2014).